RETRACTED ARTICLE: Liver X receptors constrain tumor development and metastasis dissemination in PTEN-deficient prostate cancer Advanced prostate cancer (PCa) is a clinical challenge as no curative therapeutic is available. In this context, a better understanding of metastasis and resistance mechanisms in PCa is an important issue. As phosphatase and tensin homolog (PTEN) loss is the most common genetic lesion in such cancer, we investigate human data sets for mechanisms that can constrain cancer evolution in this setting. Here we report a liver X receptor (LXR) signature, which tightly correlates with PTEN loss, in PCa. Accordingly, the LXR pathway is deregulated in prostate carcinomas in Pten -null mice. Genetic ablation of LXRs in Pten -null mice, exacerbates PCa invasiveness and metastatic dissemination, which involves mesenchymal transition and accumulation of matrix metalloproteinases. Mechanistically, PTEN deletion governed LXR transcriptional activity through deregulation of cholesterol de novo synthesis, resulting in accumulation of endogenous LXR ligands. Our study therefore reveals a functional circuit linking PTEN and LXR, and highlights LXRs as metabolic gatekeepers that are able to constrain PCa progression. Prostate cancer (PCa) is one of the most frequently diagnosed cancers in Western countries and the second leading cause of cancer death in men [1] . The clinical management of this cancer is complex, especially in the metastasic phase of the disease. Therefore, to develop effective therapeutic strategies to treat PCa and to prevent metastasic dissemination, a better understanding of metastasis and resistance mechanisms is necessary. The loss of phosphatase and tensin homolog (PTEN), which deregulates the phosphatidyl inositol 3-kinase (PI3K)/AKT pathway, is the most frequently observed mutation in PCa [2] . However, despite the high frequency of PTEN deletion in PCa, mice with intraepithelial prostate-specific deletion of Pten ( Pten pc−/− ) only recapitulate the initial phases of the human disease, but do not exhibit invasive and metastatic features [3] , [4] , [5] , [6] . This suggests the existence of adaptive responses that limit the metastatic capacity of PCa in the absence of Pten , as recently demonstrated for Smad4 [7] . It is well established that cancer cells adapt their metabolic program, in part by strongly increasing biosynthesis of key cell components in order to fuel rapid growth [8] . Accordingly, cholesterol biosynthesis, which provides an important building block for cellular membranes, is subject to reprogramming in cancer cells. There is a growing body of evidence, suggesting involvement of cholesterol metabolism in PCa, and a recent study identified an association between cholesterol ester accumulation in the prostate and increased PCa aggressiveness [9] . Cholesterol metabolism is subject to tight transcriptional and posttranscriptional regulation. The liver X receptors (LXRs), which are members of the nuclear receptor family of transcription factors, have a prominent role herein. LXRs are pivotal sensors of the cellular sterol contents owing to their ability to bind oxysterols, oxidized cholesterol derivatives and to reprogram cholesterol metabolism. Oxysterols have an established role in the prostate [10] , [11] , [12] , [13] and, accordingly, we have recently shown that both LXR isoforms (NR1H3, LXRα and NR1H2, LXRβ) protect prostatic epithelium from neoplasia in response to a high cholesterol diet [14] . In the present study, we demonstrate that LXRs constrain PTEN-dependent carcinogenesis in the prostate, and that LXR ablation in Pten pc−/− mice results in aggressive prostatic lesions associated with widespread metastatic disease. Our findings indicate that in vivo, LXRs serve a gatekeeper function to constrain prostatic adenocarcinoma in response to metabolic reprogramming of sterol metabolism by cancer cells. LXRs are gatekeepers of Pten -null prostate tumor progression We have recently reported that LXRs attenuate prostate intraepithelial neoplasia (PIN) in vivo [14] . To evaluate the status of the LXR-controlled transcriptional program in advanced prostate tumors we monitored the expression of a canonical set of LXR target genes by analyzing public datasets of human PCa collections. Unexpectedly, ONCOMINE analyses identified upregulation of the LXR transcriptional program, which was most prominent in metastatic PCa (Figs. 1a, b and Supplementary Fig. 1A ). Interestingly, evaluation of enrichment profiling (Gene Set Enrichment Analysis, GSEA) of gene sets sensitive to PTEN loss supported the existence of an inverse correlation between expression of LXR target genes and PTEN status in humans (Fig. 1c and Supplementary Fig. 1B ). We therefore decided to evaluate LXR signaling in prostate samples derived from control ( Pten pcL / L ) and prostate-specific Pten -null ( Pten pc−/− ) mice. Consistent with the finding in the human data set, levels of the established LXR targets ABCA1, FAS and APOE were substantially increased in prostates from Pten pc−/− mice (Fig. 1d, e ). Importantly, we confirmed that dysregulated LXR signaling in these mice was LXR dependent. Indeed, expression of the three LXR target genes decreased in Pten pc−/− Lxrαβ −/− mice (Fig. 1e and Supplementary Fig. 2A, B ) generated by mating of Pten pc−/− with Lxrαβ −/− mice. The effect of Pten loss on LXR signaling was not limited to ABCA1, FASN and APOE, as other LXR-regulated genes also displayed aberrant expression (Fig. 1f and Supplementary Fig. 2C, D ). Furthermore, these changes do not represent global deregulation of metabolic gene expression, as a panel of other metabolic genes remain unchanged (Fig. 1g ), and is also not the result of alterations in the expression level of Lxrα and/or Lxrβ in mouse prostates (Fig. 1h ). Fig. 1 PTEN -loss carcinogenesis is associated with transcriptional upregulation of LXR target genes. a ONCOMINE boxed plot of PTEN , FASN and APOE expression levels between human prostate gland, prostate carcinoma and metastasis in various human data sets [2] , [57] , [58] . b Heatmap of LXR target gene signature and PTEN expression in Grasso et al. [57] data set. c Gene Set Enrichment Analysis of LXR target gene signature based on PTEN status using Grasso et al. [57] data set. d HE staining and immunohistofluorescence against PTEN, AKTS473 and ABCA1 of wild type (WT) and Pten pc −/− mouse prostate tissues from 6-month-old animals. Scale bar , 100 µm. Nuclei are stained using Hoescht ( blue ). e Western blot analysis of PTEN, AKTS473, AKT, FASN, APOE and GAPDH of wild type (WT), Pten pc −/− and Pten pc −/− lxrαβ −/− mouse prostatic tissues from 6-month-old animals. f – h Relative expression of LXR targets genes, non-LXR target gene panel, Lxrα ( Nr1h3 ) and Lxrβ ( Nr1h2 ). All data are represented as mean ± SEM and statistical analyses were performed with the Student’s t -test; * p < 0.05, ** p < 0.01 and *** p < 0.001. See also Supplementary Figs. 1 and 2 Full size image To investigate the role had by LXRs in prostate carcinogenesis, we studied the consequence of their deletion in Pten pc−/− mice. Macroscopic analyses of prostates demonstrated that loss of Lxrs resulted in a marked increase in gland size and weight (Fig. 2a, b ). Importantly, Lxrαβ −/− control littermates had normal prostates, demonstrating that the loss of Lxrs is not intrinsically carcinogenic (Supplementary Fig. 3A–C ). Consistent with the prostatic phenotype, comparison of prostates from Pten pc−/− and Pten pc−/− Lxrαβ −/− mice revealed a significant increase in the frequency of invasive carcinoma both in 2- and 6-month-old mice (Fig. 2c, d and Supplementary Fig. 4A–D ). Enhanced tumor invasiveness in Pten pc−/− Lxrαβ −/− prostates was further confirmed using smooth muscle actin breakdown staining, as a proxy for tumor barrier loss (Fig. 2e and Supplementary Fig. 4E, F ). Proliferation, as assessed by Ki67 scoring, was increased in prostates of Pten pc−/− Lxrαβ −/− mice (Fig. 2f, g and Supplementary Fig. 5A–C ), as was a panel of molecular markers associated with cell cycle control and prostate homeostasis (Supplementary Fig. 5D ). In line with an increase in malignant lesions, survival of Pten pc−/− Lxrαβ −/− mice was decreased (±35%) when compared with Pten pc−/− mice (Fig. 2h ). Decreased survival prompted evaluation of the occurrence of metastasis, which is uncommon in Pten pc−/− mice. Remarkably, histopathological analysis of distant organs showed a high frequency of metastatic spread (Fig. 2i, j and Supplementary Fig. 5E ), which was confirmed by the presence of CK18- and PSCA-positive nodules in Pten pc−/− Lxrαβ −/− mouse lungs and lymph nodes (Fig. 2k ). We observed metastatic lesions in some 2-month-old Pten pc−/− Lxrαβ −/− mice that progressed to severe and systematic dissemination in 6-month-old animals (Fig. 2i and Supplementary Fig. 5F and 5G ). These observations stand in stark contrast with our observation in Pten pc−/− mice, which rarely developed metastasis before 1 year of age. Taken together, these results provide strong in vivo evidence that LXRs constrain cancer progression and dissemination in Pten pc−/− mice. Fig. 2 LXR ablation in Pten -mutant mice leads to cancer progression and metastasis dissemination. a Gross anatomy of representative prostates at 6 months of age. Seminal vesicles (SV), bladder (B), anterior prostate lobe (AP), dorso-lateral prostate lobe (DLP) and ventral lobe (VP). Scale bar , 1 cm. b Relative weight of prostates wild type (WT), Pten pc −/− and Pten pc −/− lxrαβ −/− ( N = 16/7/14). Statistical analyses were performed with the Student’s t -test. c HE-stained sections of representative dorsal prostate (DP) at 8, 11 and 20 weeks. Scale bar , 100 µm. d Histological evaluation of dorsal lobe lesions, Low-grade PIN, high-grade PIN, in situ carcinoma or invasive carcinoma. Three distant sections from each mouse (10 mice per group) were scored ( χ 2 = 17.27, p = 0.0006). e Ki67 and SMA (smooth muscle actin) immunofluorescence performed on Pten pc −/− and Pten pc −/− lxrαβ −/− prostate specimens. Acini breaks have been quantified using following criteria: discontinuous SMA staining and presence of Ki67-positive staining in surrounding stromal compartment. Nuclei are stained using Hoescht ( blue ), scale bar 100 µm. ( N = 10 per group). f Representative Ki67 immunohistochemistry on prostatic tissues from each genotype, scale bar 100 µm. g Quantification of Ki67-positive staining ( N = 8 per group). h Kaplan–Meier cumulative survival analysis showing significant decrease ( p < 0.0001) in lifespan in the Pten pc −/− lxrαβ −/− compared with Pten pc −/− group. ( N = 10/11/12). i Recapitulative table of metastatic phenotypes in Pten pc −/− and Pten pc −/− lxrαβ −/− animals. j Gross anatomy of lungs from Pten pc −/− vs. Pten pc −/− lxrαβ −/− from 6-month-old mice. k HE-stained sections and immunofluorescence detection of primary tumor site (prostate), lumbar lymph nodes and lung of Pten pc −/− and Pten pc −/− lxrαβ −/− using specific (CK18/PSCA) prostatic markers. High-magnification depicted cell arrangement within the host tissue. Scale bar , 100 µm. Nuclei are stained using Hoescht ( blue ). All data are represented as mean ± SEM. *** p < 0.001. See also Supplementary Figs. 3 , 4 and 5 Full size image PTEN deletion acts on LXR through PI3K/AKT To investigate the mechanism linking PTEN and LXRs, we took advantage of previously established immortalized cells derived from mouse prostate, mouse prostatic epithelial cells (MPECs) (Supplementary Fig. 6A, B ) [11] . As observed in vivo, expression of LXR target genes was increased in the absence of Pten in MPECs (Fig. 3a, b and Supplementary Fig. 6C ), establishing a functional link between PTEN deletion and LXR activity in tumor epithelial cells. To extend this observation to a relevant human system, we investigated LNCaP and PC3 cells, two established PTEN -negative cell lines commonly used to study PCa. First, we used LNCaP cells that have been genetically engineered to express a doxycycline-inducible PTEN–green fluorescent protein (GFP) fusion protein (LNCaP-PTEN) [15] . Remarkably, doxycycline induction leads to a marked decrease in ABCA1, APOE and FASN proteins in these cells (Fig. 3c, d and Supplementary Fig. 6D ). This effect was not limited to ABCA1 as additional LXR-regulated genes responded similarly (Fig. 3e ). To test whether the effect of PTEN on LXR signaling was dependent on its intrinsic phosphatase activity we transfected LNCaP cells with expression constructs encoding either wild type (WT) or catalytically inactive PTEN (PTEN C124A). Whereas expression of WT PTEN decreased LXR-regulated gene expression, the catalytic mutant failed to do so (Fig. 3f and Supplementary Fig. 6E ). Accordingly, transfection of mutant PTEN did not reduce the level of APOE and FASN protein in these cells (Fig. 3g ). Similar results were obtained using PC3 cells, a second PTEN-negative cell line (Supplementary Fig. 6F–H ). Collectively, these results demonstrate that PTEN’s intrinsic phosphatase activity is an important determinant of LXR signaling. As PTEN is a key regulator of PI3K/AKT signaling [16] , we reasoned that this signaling pathway may couple PTEN and LXRs. Consistent with this idea, LNCaP and PC3 cells treated with two PI3K inhibitors, Wortmannin and LY294002, exhibited decreased expression of LXR target genes (Fig. 3h, i and Supplementary Fig. 7A–D ). To further substantiate the role of PI3K/AKT in regulating LXR signaling, we made use of a dominant negative AKT construct. Similar to the PI3K inhibitors, this genetic manipulation decreased expression of LXR target genes in both cell lines (Fig. 3j and Supplementary Fig. 7E–G ). Reciprocally, we reasoned that forced activation of PI3K/AKT-dependent signaling in PTEN-positive cells should increase LXR pathway. To test this notion, we expressed a constitutively active form of AKT (MyrAKT) or of the PI3K catalytic subunit p110 (p110CAAX) in PTEN-positive DU145 cells. As posited, this resulted in a substantial increase in LXR signaling (Fig. 3k, l and Supplementary Fig. 7H ). Therefore, our pharmacologic and genetic experiments substantiate a key role of the PTEN/PI3K/AKT axis in regulating LXR signaling in prostate epithelial cells. Fig. 3 PTEN -status controls LXR activities in PCa cells through PI3K/AKT pathway. a Relative expression levels of Abca1 , Abcg1 , Idol , Fasn and ( b ) PTEN, AKTS473, AKT, FASN and β-ACTIN protein accumulation levels in MPECs (mouse prostatic epithelial cells) wild-type ( + / + ) and Pten −/− . c Immunofluorescence of PTEN–GFP and ABCA1 in LNCaP-PTEN inducible cell line treated with DMSO or Doxycycline (25 µM). Nuclei are stained using Hoescht ( blue ). Scale bar : 100 µm. d Quantitative measurement of ABCA1-positive cells has been performed. e Relative expression of LXR target genes in LNCaP-PTEN-inducible cell line treated with DMSO or Doxycycline (25 µM). f , g Relative gene expression analysis and protein accumulation of LXR targets in LNCaP cells transfected with PTEN and PTENC124A expression construct vs. empty vector. h , i Relative expression and protein accumulations of LXR targets in LNCaP cells treated with PI3K inhibitors Wortmannin (0.5 µM) or LY294002 (20 µM). j Relative accumulation of ABCA1 , ABCG1 , FASN and IDOL in LNCaP cells transfected with AKTd/n (dominant-negative) expression vector. k Immunofluorescence against AKTS473 and ABCA1 in DU145 transfected with myrAKT or p110CAAX (dominant-positive) expression vectors. Nuclei are stained using Hoescht ( blue ). Scale bar : 100 µm. l Relative accumulation of ABCA1 , ABCG1 , FASN and IDOL in DU145 transfected with myrAKT of p110CAAX expression vectors. m Luciferase activity measurement in MEF Pten −/− transfected with 3xLXREtk-Luc reporter construct or tk-Luc construct as a control and with PTEN and PTENC124A expression construct versus empty vector. n Luciferase activity measurement in MEF + / + , Lxr α −/− , Lxr β −/− or Lxr αβ −/− transfected with 3xLXREtk-Luc reporter construct and expression vector encoding myrAKT. T0901317 (1 µM) treatment has been performed as a control. MEF Lxr αβ −/− were rescued using LXRα and LXRβ expression vectors. o Abca1 and Fasn relative expression in MPEC Pten −/− and Pten −/− lxrαβ −/− treated with Wortmannin (0.5 µM), LY294002 (20 µM) and/or T0901317 (1 µM). For whole experiments, the results represent the means ± SEM of three independent experiments; * p < 0.05; ** p < 0.01; *** p < 0.001. See also Supplementary Figs 6 and 7 Full size image To establish that regulation of LXR signaling by PTEN involves modulation of their transcriptional activity we introduced an LXRE-driven reporter construct in Pten −/− mouse embryonic fibroblasts (MEFs). In line with our earlier observations in the prostate-derived cell lines, PTEN expression decreased the LXR-reporter signal in an activity-dependent manner, as this was not observed when a PTEN C124A mutant was introduced (Fig. 3m and Supplementary Fig. 7I ). We therefore conclude that PTEN loss induces expression of LXR target genes by regulating LXR’s transcriptional activity. LXRs have been previously reported to act as tumor suppressors in melanoma, in which LXRβ seems to be the prominent LXR isoform [17] . Unlike melanoma, in prostate tumors both LXR isoforms are expressed [14] . To address whether one of the isoforms is specifically PTEN responsive, we studied MEFs from single and double LXR knockout mice (Fig. 3n ). To this we transfected the MEFs with MyrAKT, a constitutively active AKT construct, to mimic PTEN loss. We observed that only loss of both LXR isoforms render the cells insensitive to constitutive activation of the PI3K/AKT pathway, indicating that with respect to PTEN the two isoforms are redundant. Several potential molecular mechanisms may underlie modulation of LXR transcriptional activity. One plausible possibility is that PTEN prevents production of endogenous LXR ligands, and that when expressed, the absence of these ligands attenuates LXR signaling. To test this idea we inhibited PI3K using Wortmannin and LY294002 in Pten −/− MPECs resulting in a decreased Abca1 and Fasn expression. Importantly, expression of these genes could be fully restored by treating the cells with the synthetic LXR ligand T0901317, in an LXR-dependent manner (Fig. 3o and Supplementary Fig. 7J, K ). Taken together, these findings suggest that PTEN expression influences LXR signaling in PCa through a PI3K/AKT-dependent pathway, and that this may impinge on tumor sterol metabolism and generation of endogenous LXR ligands. PTEN deletion drives LXR activation through cholesterol We next sought out to determine how the PTEN/PI3K/AKT axis modulates LXR activity in PCa. Based on our experiments with the synthetic LXR ligand we postulated that this might be mediated by the production of endogenous LXR ligands (e.g. oxysterols) and tested this by determining the hydroxycholesterol species present in prostates of WT and Pten pc−/− mice focusing on established LXR ligands [18] . We observed that the levels of 5,6β-epoxy-cholesterol and 5,6α-epoxy-cholesterol, but not 22(R)-hydroxycholesterol and 27-hydroxycholesterol, (27-OHC) were significantly increased in Pten pc−/− prostates (Fig. 4a and Supplementary Fig. 8A ). Reciprocally, transfection of PTEN or a AKTd/n expression constructs into PC3 PTEN-negative cells significantly decreased 5,6β-epoxy-cholesterol and 5,6α-epoxy-cholesterol accumulation (Fig. 4b and Supplementary Fig. 8B ). Similarly, accumulation of 22(R)-hydroxycholesterol and 27-hydroxycholesterol were also slightly reduced as a result of this treatment. Together, these findings pointed out 5,6α-epoxy-cholesterol as a putative endogenous LXR ligand in mouse prostates as previously reported by Berrodin et al. in keratinocytes [19] . In order to confirm that PTEN governs the production of endogenous LXR ligands, we induced PTEN expression in LNCaP doxycycline-inducible cells. Consistent with reduced production of endogenous ligands, the level of ABCA1 protein decreased (Fig. 4c ). However, after treating PTEN-induced cells with T0901317, the level of Abca1 , as well as others LXR target genes was fully restored (Figs. 4c, d ). This finding corroborates data from MPECs and showed that intrinsic LXR signaling was unaltered in PTEN positive cells, but that ligand availability may be the limiting factor. Consistent with this, T0901317 also abolished repression of LXR signaling by PI3K inhibitors in LNCaP and PC3 cells (Supplementary Fig. 8C, D ). Fig. 4 PTEN -loss results in an accumulation of sterols. a Levels of 5,6β-epoxy-cholesterol, 5,6α-epoxy-cholesterol, 22(R)-hydroxycholesterol and 27-hydroxycholesterol in prostatic samples from wild type (WT) ( N = 4) and Pten pc −/− mice ( N = 5). b Levels of 5,6β-epoxy-cholesterol, 5,6α-epoxy-cholesterol, 22(R)-hydroxycholesterol and 27-hydroxycholesterol in PC3 cells transfected with PTEN expression construct vs. empty vector. c , d Immunofluorescence of PTEN–GFP and ABCA1 proteins, and relative expression of LXR target genes in LNCaP-PTEN-inducible cell line treated with DMSO or Doxycycline (25 µM) with or without T0901317 (1 µM). Nuclei are stained using Hoescht ( blue ), scale bar 100 µm. e Luciferase activity measurement in wild type MEF transfected with Gal4-LXRαLBD or/and Gal4-LXRβLBD and UAS-Luciferase after incubation with medium conditioned during 24 h by PC3 cells transduced with SULT2B1b or Mock construct. FBS and T0901317 are used as controls. f LXR target genes expression in PC3 cells transduced with SULT2B1b or Mock construct. g Luciferase assays in wild type MEF transfected as indicated above after incubation with medium conditioned during 24 h by PC3 cells transfected with PTEN, PTENC124A or AKTd/n expression construct versus empty vector. FBS and T0901317 are used as controls. For experiments b – g , data are the result of three independent experiments. All the statistical analyses were performed with the Student’s t -test and are represented as mean ± SEM; * p < 0.05; ** p < 0.01; *** p < 0.001. See also Supplementary Figs. 8 , 9 and 10 Full size image To definitively demonstrate that PTEN status governs production of oxysterols, we tested whether PC3 culture supernatants (i.e., conditioned medium) contain LXR agonists, by determining whether the supernatants can induce expression of a an LXR reporter system (Gal4-LXRαLBD, Gal4-LXRβLBD and UAS-Luc) reconstituted in MEFs (Fig. 4e ). We found that supernatants from PC3 cells transduced with a virus encoding SULT2B1b , a LXR agonist-inactivating enzyme [20] , [21] , [22] , [23] resulted in a marked decrease of LXR transcriptional activity monitored either using the supernatant assay (Fig. 4e and Supplementary Fig. 8E ) or when directly measuring target gene expression (Fig. 4f ). Similarly, PTEN or AKTd/n transfected PC3 cells exhibited lower induction of LXRα and LXRβ transcriptional activity (Fig. 4g ). These experiments support the notion that PI3K activity is associated with the production of endogenous LXR agonists, and that therefore an important consequence of PTEN loss is enhanced LXR signaling. Oxysterols originate from both enzymatic activity and lipoperoxidation, and we therefore aimed to identify the source of the elevated LXR ligands produced as a result of PTEN loss. Analysis of PTEN-null prostates revealed increased expression of Cyp46 and Cyp7a1 , yet the level of the corresponding products of these enzymes was not elevated (Supplementary Fig. 9A ). This finding indicate that 5,6α-epoxy-cholesterol could be produced from cholesterol by an unidentified cytochrome P450. Such stereospecific transformations have already been reported in the microsomal fraction of the bovine adrenal cortex [24] . To evaluate the role of lipoperoxidation we tested whether vitamin E, a potent inhibitor of this process that also blocks cholesterol epoxidation, altered the PTEN-dependent LXR response. This may be particularly relevant, as 5,6β-epoxy-cholesterol and 5,6α-epoxy-cholesterol represent major accumulating sterol species in Pten pc−/− prostates (Fig. 4a ). Treating cells with vitamin E decreased expression of LXR target genes in PTEN-negative cell lines (Supplementary Fig. 9B, C ) and limited LXR activation in the supernatant assay (Supplementary Fig. 10A, B ). Our results suggest that lipoperoxidation participate, at least in part, to LXRs activation when PTEN is lost. Another source of increased oxysterols and LXR ligands in Pten pc−/− prostates may be a result of increased de novo cholesterol synthesis, as previously proposed in human-derived prostate cell lines [25] , [26] , [27] . To test this hypothesis, we determined the expression of genes in the SREBP2-regulated cholesterol synthesis pathway. Our analysis revealed a marked increase in expression of SREBP2-regulated genes and of SREPB2 itself (Fig. 5a ). Furthermore, the levels of cholesterol biosynthesis intermediates and cholesterol were also elevated (Fig. 5b ). Notably, we also detected marked elevation of desmosterol, a potent endogenous LXR ligand [28] . We next reasoned that if enhanced cholesterol synthesis drove LXR signaling in PTEN -null tumors, this process should be sensitive to inhibition by statins that block HMGCoA reductase, a rate-limiting step in cholesterol biosynthetic pathway. As expected, simvastatin treatment increased expression of HMGCR in LNCaP cells (Fig. 5c ) and reciprocally repressed both ABCA1 and FASN expression in LNCaP cells (Fig. 5c and Supplementary Fig. 11A ), as well as in PC3 cells (Supplementary Fig. 11B ) and MPECs (Supplementary Fig. 11C ). Repression of LXR pathway by statins could be completely overcome by T0901317 treatment (Fig. 5c and Supplementary Fig. 11A–C ), consistent with the idea that de novo synthesis was responsible for the production of endogenous LXR ligands in response to PTEN loss. To conclusively demonstrate that reduced endogenous LXR ligands production in PTEN-null cells was the underlying cause for decreased LXR signaling following statin treatment, we blocked HMGCR with simvastatin and supplemented culture medium with a high concentration of mevalonate, the product of HMGCR activity. As expected, mevalonate overcame inhibition of de novo synthesis by simvastatin, restored metabolic pathway and expression of ABCA1 (Fig. 5d ). Restoration of ABCA1 and FASN expression by exogenous mevalonate was dose-dependent (Fig. 5e ) and was mirrored by a corresponding decline in HMGCR expression. Thus, having established that altered production of endogenous ligands underlay the effect of PTEN on LXRs, we reasoned that SREBP2, the master transcriptional regulator of cholesterol synthesis, is sensitive to the PTEN status. To evaluate activity of the SREBP2-regulated pathway we monitored the processing of SREBP2 into the transcriptional active “mature” form and the levels of the SREBP2 canonical targets, HMGCR and SQLE . Pharmacological inhibition of PI3K in LNCaP cells markedly decreased SREBP2 processing and the protein levels of HMGCR and SQLE (Fig. 5f ). Similar results were obtained in PC3 cells using PI3K inhibitors (Supplementary Fig. 11D ) and by overexpression of a dominant-negative AKT expression construct (Supplementary Fig. 11E ). Interestingly, restoration of de novo synthesis by exogenous mevalonate in PC3 cells in the context of PI3K inhibition increased ABCA1 but also the levels of APOE, another LXR target (Fig. 5g ). Finally, SREBP2 knockdown in PC3 cells resulted in a significant decrease of SREBP2 and LXR target genes expression (Fig. 5h ) and in the ability of PC3 supernatants to induce LXR transcriptional activity (Supplementary Fig. 11F ). Cumulatively, these experiments support the idea that the PI3K pathway controls LXR signaling by controlling production of endogenous ligand through cholesterol de novo synthesis. To test this idea in vivo, we orally administered simvastatin to Pten pc−/− mice. This treatment suppressed accumulation of both Fasn and Abca1 at the messenger RNA level and protein level (Figs. 5i, j ), which was not observed in MPECs derived from Pten pc−/− Lxrαβ −/− prostates (Supplementary Fig. 11C ). Simvastatin treatment not only blocks LXR activation in the absence of PTEN but also dramatically decreases cholesterol supply from de novo synthesis. Consistent with the role of cholesterol in tumor growth, simvastatin treatment was associated with a decrease in tumor progression and proliferation in Pten pc−/− mice (Supplementary Fig. 12A–E ). Therefore, PTEN inactivation in PCa cells results in increased cholesterol de novo synthesis, which results in increased production of endogenous LXR ligands and altered sterol balance in tumor tissue. Fig. 5 PTEN -loss results in an increased cholesterol de novo synthesis. a Relative accumulation of Srebp2 , Hmgcr , Sqs and Hmgcs1 transcripts in prostate of wild type (WT) and Pten pc −/− mice. ( N = 10 per group). b Accumulation of cholesterol precursors, lanosterol, lathosterol, desmosterol and cholesterol in prostatic samples from wild type (WT) ( N = 4) and Pten pc −/− mice ( N = 5). c qPCR analysis of HMGCR , ABCA1 and FASN expression in LNCaP cells treated with Simvastatin (2,5 µM) alone or with T0901317 supplementation (1 µM). Experiments have been performed in three experimental replicates. d qPCR analysis of ABCA1 and HMGCR expression in LNCaP cells treated with Simvastatin (2,5 µM) alone or with mevalonate (500 µM). e qPCR analysis of HMGCR , ABCA1 and FASN expression in PC3 cells treated with LY294002 (20 µM) alone or with increasing amounts of mevalonate (100 µM, 500 µM, 1 mM, 10 mM). f Western blot analysis of SREBP2 cleaved form, HMGCR and SQLE respective accumulation in LNCaP cell line. AKTS473 is used to confirm Wortmannin and LY294002 treatment efficiency and β-ACTIN as a loading control. g Western blot analysis of HMGCR, SQLE and APOE in PC3 cells treated with LY294002 (20 µM) alone or in combination with mevalonate (500 µM). AKTS473 and AKT are used to confirm Wortmannin and LY294002 treatment efficiency and β-ACTIN as a loading control. h SREBP2 and LXR target genes expression in PC3 cells transfected with siSREBP2 or siGFP as control. Experiments have been performed in three experimental replicates. i Relative expression of Hmgcr , Abca1 and Fasn on prostate samples from wild type mice and Pten pc −/− mice treated with vehicle (methylcellulose) or Simvastatin (40 mg kg −1 ). j Immunofluorescence detection of FASN and ABCA1 on prostate samples from wild type mice and Pten pc −/− mice treated with vehicle (methylcellulose, N = 6) or Simvastatin (40 mg kg −1 , N = 6). Nuclei are stained using Hoescht ( blue ), scale bar 100 µm. k qPCR analysis of Abca1 and Fasn expression on MPEC Pten −/− or Pten −/− lxrαβ −/− treated with simvastatin alone (2,5 µM) or in combination with T0901317 (1 µM), N = 3 per group. All data are represented as mean ± SEM and statistical analyses were performed with the Student’s t -test; * p < 0.05; ** p < 0.01; *** p < 0.001. See also Supplementary Figs. 11 and 12 Full size image LXRs control tumor invasiveness and metastatic spread The dramatic growth of Pten pc−/− adenocarcinomas when Lxrs were genetically ablated, and particularly the high penetrance of metastatic disease in this model, prompted evaluation of the role of LXRs in the control of carcinogenic invasiveness. In order to identify the underlying molecular mechanisms, we conducted a transcriptomic analysis of WT, Lxrαβ −/− , Pten pc−/− and Pten pc−/− Lxrαβ −/− prostate samples (Supplementary Fig. 13A–C ). GSEA analysis of transcriptomic data identified epithelial–mesenchymal transition (EMT) as the most deregulated pathway in Pten pc−/− Lxrαβ −/− compared with Pten pc−/− prostates, consistent with the high occurrence of metastasis following inactivation of both Pten and Lxrs . Further analysis of the EMT markers Zeb1 , Twist1 , Twist2 , Snai1 and Vimentin between revealed that loss of Lxrs in the context of Pten inactivation resulted in enhanced expression of these markers, consistent with a switch from epithelial to mesenchymal identity (Figs. 6 a-c). Further consistent with the EMT phenotypic shift, the Ncad / Ecad ratio was inverted in Pten pc−/− Lxrαβ −/− prostate tumors (Figs. 6a, b ). Another well-established determinant that supports tumor aggressiveness is the overexpression of matrix metalloproteinases (MMPs), which allow cells to efficiently degrade the surrounding matrix and migrate. Accordingly, we found enhanced expression of Mmp1 , Mmp2 , Mmp7 and Mmp9 (Fig. 6d ), and significant accumulation of MMP9 protein in Pten pc−/− Lxrαβ −/− prostates (Fig. 6e ). In contrast, expression of Timp2 , an endogenous inhibitor of MMPs, was decreased (Fig. 6d ). Furthermore, immunostaining of metastasis in lungs of Pten pc−/− Lxrαβ −/− revealed extensive MMP9 signal at the interface between metastatic cells and the pulmonary matrix (Fig. 6f ). This demonstrates the invasive properties of metastatic cells within the lung. Fig. 6 LXRs control invasiveness of tumor cells through upregulation of EMT and metalloproteases. a , b Relative expression and protein accumulation of EMT markers in prostate from wild type (WT), Pten pc −/− and Pten pc −/− lxrαβ −/− mice ( N = 10/7/8). c Immunofluorescence staining against EMT markers VIMENTIN and SNAI, together with Ki67. Nuclei are stained using Hoescht ( blue ). d Relative expression analysis of metalloproteinase genes Mmp1, 2, 7, 9 and negative regulator Timp2 in prostate from wild type (WT), Pten pc −/− and Pten pc −/− lxrαβ −/− mice ( N = 10 per group). e MMP9 protein accumulation in prostate from wild type (WT), Pten pc −/− and Pten pc −/− lxrαβ −/− mice. f Histological and immunofluorescence staining for MMP9 in lung from Pten pc −/− and Pten pc −/− lxrαβ −/− mice. White arrows indicate the positive MMP9 staining surrounded metastatic cells in contact with matrix. Asterisks identify metastatic cells and black arrows the surrounded pneumocytes. Nuclei are stained using Hoescht ( blue ). All data are represented as mean ± SEM and statistical analyses were performed with the Student’s t -test; ** p < 0.01; *** p < 0.001. See also Supplementary Fig. 13 Full size image Our results clearly demonstrate that LXRs can constrain PCa metastatic spread in vivo. However, in our model LXRs are inactivated in all cells of the body. Therefore, metastatic spread could be the result of LXRs inactivation within epithelial cells, their microenvironment or both. To investigate the epithelial cell-autonomous effects of Lxr inactivation, we first tested the ability of PC3 cells transduced with SULT2B1b to migrate across a matrix, using Boyden chambers (Fig. 7a ). Consistent with a direct role of LXRs within epithelial cells, PC3 cells that overexpressed SULT2B1b showed a greater capacity to migrate throughout the matrix. In aggregate with our earlier results, this suggests that oxysterol production, and as a result LXR activation, act to limit PC3 invasiveness in vitro. To address whether this is also the case in vivo, we could not use the Pten pc−/− Lxrαβ −/− , as these harbor a global loss of LXR that does not allow the isolated study of prostate cells. As an alternative, we therefore evaluated metastatic dissemination in immune-deficient mice that were implanted with prostate tumors originating from Pten pc−/− and Pten pc−/− Lxrαβ −/− (Fig. 7b ). Consistent with data in the genetic models, Pten pc−/− Lxrαβ −/− implants exhibited a higher proliferation rate than Pten pc−/− implants (Figs. 7c, d ). Importantly, metastatic dissemination to peripheral organs was only observed in mice implanted with Pten pc−/− lxrαβ −/− tumors with a 100% penetrance (Figs. 7e, f ). Therefore, our results strongly support the idea that the tumor-suppressive activity of LXRs in PCa is cell autonomous and is the result of altered cellular cholesterol metabolism. Fig. 7 LXRs downregulate intrinsic invasiveness properties of PTEN-negative tumor cells. a Boyden chamber assays performed using PC3 cells transduced with SULT2B1b or Mock construct. Migrated cells are stained with hematoxylin staining ( N = 8), scale bar 100 µm. b Description for renal subcapsular implantation in immunocompromized host mice (Nude mice) of prostate specimen from Pten pc −/− and Pten pc −/− lxrαβ −/− mice. c , d Representative histological features (HE) and Ki67 staining of implant after 1 month of growth, and quantification of Ki67-positive cells from Pten pc −/− ( N = 6) and Pten pc −/− lxrαβ −/− ( N = 6) grafts on Nude mice, scale bar 100 µm. e Evaluation of metastatic dissemination on lumbar lymph nodes and lung using prostatic markers CK18 and PSCA in grafted nude mice ( N = 6 per group). Nuclei are stained using Hoescht ( blue ), scale bar 100 µm. f Recapitulative table of metastatic phenotype in lungs and lumbar lymph nodes of grafted Nude mice. All data are represented as mean ± SEM and statistical analyses were performed with the Student’s t -test; *** p < 0.001 Full size image Management of advanced PCa requires a better understanding of the molecular mechanisms influencing development, progression and eventual metastasis in order to identify tractable therapeutic targets. The most important aspect of our work is the finding of a functional interaction between PTEN and LXRs. Specifically, we demonstrate that PTEN loss, the most frequent genetic alteration observed in human PCa, is associated with increased activation of the LXR transcriptional pathway. Accordingly, combined ablation of both Lxr isoforms and Pten in mouse prostates led to a dramatic increase in prostate carcinoma invasiveness and associated metastatic dissemination. These findings highlight the crucial protective role of LXRs during prostate carcinogenesis. The molecular mechanism sustaining this deregulation involves enhanced activation of the PI3K/AKT pathway. Altered signaling of this pathway leads to aberrant LXR activation as a result of excessive production and accumulation of endogenous ligand and, in line with this, inhibition of the mevalonate pathway by blocking de novo cholesterol synthesis decreases LXR target gene expression and reduces tumor aggressiveness in vivo. Taken together, our study identifies LXRs as an important determinant of PCa in the setting of PTEN loss owing to their ability to suppress tumor invasiveness and dissemination. Altered cholesterol metabolism is emerging as a metabolic signature of cancer cells. In 1942, accumulation of cholesterol was already reported in adenomas of enlarged prostates [29] . This finding has been overlooked for a long time and viewed as a secondary metabolic adaptation of PCa tumors. This point of view has recently been challenged by several studies [27] , [30] and, notably, accumulation of cholesterol esters in lipid droplets induced by PTEN loss is now recognized as a hallmark of PCa aggressiveness [9] . Accordingly, manipulations leading to the depletion of cholesterol-ester storage result in reduced PCa invasiveness, highlighting the importance of cellular mobilization of cholesterol as a powerful driver of tumor aggressiveness. In line with this idea, metabolomic analysis of PCa metastasis revealed significant accumulation of cholesterol that was also associated with high levels of the LDLR [30] . Together with our data, these findings emphasize the association between cholesterol accumulation and metastatic processes, as we are also reporting herein. The molecular mechanisms governing tumor cholesterol homeostasis in PCa are, however, less clear. The autonomous capability of cells to ensure cholesterol de novo synthesis in response to PTEN loss warrants re-evaluation of the classical paradigm of cholesterol homeostasis regulation. Indeed, PCa cells exhibit an increase in both expression and cleavage of SREBP2, a transcription factor that controls the cholesterogenic program, with a concomitant accumulation of hydroxycholesterol species. Studies conducted on LNCaP and PC3 cell lines showed that sterol sensing and the cholesterol-dependent control of SREBP2 cleavage is impaired, which results in deregulation of metabolic feedback of this pathway. This concept is consistent with the accumulation of cholesterol observed in clinical PCas samples [31] . As a possible explanation for deregulated cholesterol synthesis in PCa, AKT and downstream mTORC1 signaling have been shown to have a prominent role in regulating the activation of the SREBP-controlled cholesterogenic program [32] , [33] . Taken together, these reports point toward a mechanism by which PCa cells are able to maintain cholesterol de novo synthesis and uptake fully active for enhanced proliferation. In the setting of enhanced SREBP2 activation and cholesterol production, LXRs could represent a defense mechanism to limit cellular cholesterol accumulation and to suppress tumor progression. Under these conditions, LXRs are activated by a specific panel of “LXR-agonists” oxysterols and/or some intermediates of the cholesterol biosynthetic pathway, such as desmosterol [28] . This promotes cholesterol efflux [34] and limits further accretion of lipoprotein-derived cholesterol [35] . Interestingly, a similar idea was recently put forward to explain how LXRβ  may limit dissemination of melanoma [17] . In our study, we showed that LXR endogenous ligand accumulation in response to PTEN loss results in suppression of invasion and metastasic spreading of PCa. Whether this is dependent on a specific LXR-regulated gene or the result of the combinatorial effect of LXR activation remains unknown so far. It is interesting to note that in melanoma, induction of ApoE expression both in tumor and stromal cells seems to explain, at least in part, the effect of LXR activation [17] . Beyond its role in transporting cholesterol, ApoE can also bind LRP1 and LRP8 on tumor and endothelial cells, respectively, and thus constrain cancer cell invasion and endothelial recruitment. Whether this underlies the effect of LXRs in PCa remains to be studied. However, other LXR target genes may also underlie the suppressive activity of LXRs during prostate carcinogenesis. For example, induction of the cholesterol efflux transporter ABCG1 by LXR agonists has been shown to attenuate signaling pathways emanating from lipid rafts, and specifically the PI3K pathway in LNCaP cells [13] . Thus, loss of LXRs in vivo may result in enhanced pro-oncogenic signaling from lipid rafts to facilitate cancer promotion. Clearly, identification of the bona fide LXR target gene(s) able to constrain PTEN -driven carcinogenesis is an important issue. This could allow better understanding of the link between cholesterol homeostasis and carcinogenic processes, and could provide new target(s) for alternative therapeutic strategies to treat advanced PCa. Despite compelling evidence for their antitumor activity [10] , [12] , [13] , [14] , the roles of LXRs in tumors in general, and more specifically in PCa, are not well defined. Although we clearly demonstrate that LXRs control intrinsic invasiveness properties of epithelial prostate tumor cells using implanted grafs in athymic mice, one cannot rule out an important role for LXRs in the tumor microenvironment. In this setting, Villablanca et al. [20] have reported that production of LXR ligands by various tumor cells impairs dendritic cell recruitment through inhibition of CCR7, which inhibits immune cells antitumor response. This observation is supported by a study reporting that 27-OHC, an established LXR ligand, activates LXR and promotes metastatic dissemination in breast cancer [36] . Interestingly this effect on dendritic cells is not observed in vivo in colon cancer [37] , clearly demonstrating that the role of LXRs in cancer is likely to be tumor-type specific. Overall, distinct pro- and anti-tumor effect of cholesterol metabolites should be carefully addressed given there are dependent of various parameters such as cell compartment, cancer type and enzymatic environment [38] , [39] . Interestingly, dendrogenin A, an enzymatic product of 5,6α-epoxycholesterol conjugated with histamine exhibits re-differentiation and growth control properties that improved animal survival [40] . A parallel between the present report and dendrogenin A effects highlight that a better understanding of metabolic branches of cholesterol together with LXR signaling activity is a key point in cancer biology. In PTEN-null adenocarcinomas, the origin of 5,6α-epoxycholesterol is still unclear. 5,6α-Epoxycholesterol could be metabolized by different enzymes to other active metabolites that may modulate LXR activities. Indeed, the 3β-sulfated form of 5,6α-epoxycholesterol and also 7-ketocholesterol produces antagonist ligands of the LXRs [41] . Moreover, 3β-sulfated 5,6α-epoxycholesterol is a transcriptional modulator of the LXRβ in breast cancer cells and mediates the LXRβ-dependent cytotoxic activity of molecules used in the clinic for breast cancer treatment such as Tamoxifen [42] . Finally, LXR agonist production in PTEN-null cancer cells results partly from lipoperoxidation as emphasized by vitamin E supplementation experiments. These findings indicate that the redox status of cancer cells in absence of PTEN needs to be considered with respect to LXR signaling activity. Our results also show that LXR activation is associated with the control of EMT in Pten -mutant tumor cells. These observations are in agreement with accumulation of SNAIL in Lxrαβ −/− mouse prostate as reported by Kim et al. [43] in benign prostate hyperplasia. In combination with a PTEN mutation, in vivo genetic ablation of LXRs increases EMT and thus facilitates progression of prostatic carcinoma towards metastasis. Nevertheless, how LXRs control gene expression involved in the EMT process remains unclear. One possibility, alluded to above, is that this could be the result of altered lipid-raft-derived signaling in the absence of LXRs. Supporting this hypothesis, cholesterol medium enrichment increases accumulation of transforming growth factor-β (TGFβ) receptors in rafts and enhances their downstream signaling [44] . Conversely, cholesterol lowering/depleting agents may change the binding ratio of TGFβ to TGFβ-RII and -RI, which critically balances activity of this pathway. We thus speculate that absence of LXRs may increase cholesterol accumulation in lipid rafts, and that this in turn can stimulate TGFβ and downstream Smad signaling resulting in enhanced EMT, as we observe in Pten pc −/− Lxrαβ −/− prostates. Collectively, this study highlights LXRs as potent tumor suppressors in PCa and as a key determinant of prostate carcinogenesis and metastatic spread. Their effect is maintained by a marked metabolic shift in Pten -null PCa cells involving enhanced cholesterol biosynthesis. These findings support the development of therapeutic strategies that target cholesterol metabolism, next to currently established treatment modalities that target androgen receptor signaling. Given their ability to limit metastatic spread, LXRs are potential therapeutic targets in metastatic PCa, and that we need to reconsider the use of LXR agonists despite their side effects such as hypertriglyceridemia. Combining hormonal treatment agents with LXR ligands could represent a promising approach to treat metastatic PCa, which warrants further study. Animals experiments All mouse studies were conducted according to standard handle and care in agreement with the local ethic committee C2E2A. For simplicity, PB-cre4 +/+ :Pten loxP/loxP are referred as WT and PB-cre4 T/+ :Pten loxP/loxP as Pten pc −/− . Pten pc −/− mice were provided by NCI mouse repository [6] , [45] , [46] . Lxrα −/− :Lxrβ −/− mice were obtained from Dr. David Mangeldorf’s Lab (University of Texas Southwestern, Dallas, TX). Pten loxP/loxP :PB-cre T/+ :lxrα −/− :lxrβ −/− were named Pten pc −/− Lxrαβ −/− and obtained by breeding the two lastest transgenic strains. Pten loxP/loxP :PB-cre +/+ :Lxrα −/− :Lxrβ −/− control littermates as referred as Lxrαβ −/− in the manuscript. For simvastatin treatment experiments, mice were gavaged methylcellulose or simvastatin (Sigma-Aldrich) at 40 mg kg −1 three times a week during 1 month. For subrenal grafting experiments, 2-month-old athymic nu/nu mice (Charles River) were used. Dorsal prostates of Pten pc −/− and Pten pc −/− Lxrαβ −/− aged of 6 months were collected and then freshly grafted under the renal capsule of anesthetized male nude mice. After prostate implantation and kidney repositioning, mice were sutured on skin and muscle planes. Prostatic grafts were collected 1 month later. Lung and lumbar lymph nodes were analyzed for metastasis development by hematoxylin/eosin coloration and immunohistochemistry. Reagents T0901317 ligand was purchased from Cayman Chemical (71810). Simvastatin (S6196), Doxycycline (D9891) and Vitamine E (T3376) were purchased from Sigma-Aldrich, Wortmannin (#9951) and LY294002 (#9901) from Cell Signaling Technology. Most of the reagents were used in the cell culture diluted in DMSO (Sigma-­Aldrich). Primary and secondary antibodies used in immunoassay and western blot are listed in Supplementary Tables 1 and 2 . Cell culture, treatments, viral production and transfection All cell lines were cultured at 37 °C in 5% CO 2 atmosphere. LNCaP, PC3 and DU-145 cell lines were kindly provided by Professor Guido Verhoeven and Professor Franck Claessens, and LNCaP-PTEN inducible cell line by Professor Jan Trapman and Professor Guido Jenster. MPEC and MEF cells have been established in the lab. LNCaP and PC-3 cells were grown in RPMI-1640 medium (Invitrogen), and DU145 and MEFs in DMEM medium (Invitrogen), containing penicillin/streptomycin (100 mg ml −1 ), l -glutamine (2 mM) and supplemented with 10% fetal bovine serum (FBS) (Biowest). LNCaP-PTEN cell line stably transfected with TET-ON vector (van Duijn et al. [15] ) was cultured in RPMI-1640 medium containing penicillin/streptomycin (100 mg ml −1 ), supplemented with 5% tetracyclin-free FBS (Biowest), neomycin (800 μg ml −1 ) and zeocin (200 μg ml −1 ). Transfections were performed using jetPRIME (PolyPlus transfection) according to the manufacturer’s informations in 10% FBS-supplemented medium. Treatments were performed in 2% Lipoprotein-deficient serum (LPDS) during 24 h. pCMV6-HA-myrAKT and pCMV6-HA-AKTd/n were kindly provided by Dr. Nahed N Ahmed [47] . pcDNA3-p110CAAX was kindly provided by Dr. Julian Downward [48] . pGFP–PTEN and pGFP–PTEN C124A vectors were obtained from Addgene (Tamura et al. [16] ). pCMX-mLXRα and pCMX-mLXRβ have been kindly provided by David Mangelsdorf [49] . SULT2B1b-expressing cell lines were derived by transduction of the PC3 cells with the retroviral vector LSULTB1bSΔN coding for the mouse SULTB1b gene and for the cell surface marker LΔNGFr as already described [20] , [50] . Tumor cell lines were infected by the exposure to virus-containing supernatant in the presence of 8 µg ml −1 of polybrene. Transduction efficiency was measured by fluorescence-activated cell sorting analysis for LNGFr expression. RNA interference was employed to specifically deplete endogenous SREBP-2 with the targeting sequence 5′-CAACAGACGGUAAUGAUCACGUU-3′. RNA interference directed against GFP was used as control 5′-ACUACCAGCAGAACACCCCUUUU-3′. Transfections were performed using jetPRIME as described above. Quantifications or representative pictures represent, at least, three independent experiments. Invasion assays Invasion analyzes were performed using Boyden chambers (Millipore) with 8 µm pore-sized membranes, coated with Matrigel (BD Bioscience). PC3-mock (2.5 × 10 5 ) or transduced with lentivirus encoding SULT2B1b cells were seeded in the upper chamber in minimum medium RPMI-1640 medium (Invitrogen) containing penicillin/streptomycin (100 mg ml −1 ) and l -glutamine (2 mM). The lower chamber contains RPMI-1640 medium (Invitrogen) supplemented with penicillin/streptomycin (100 mg ml −1 ), l -glutamine (2 mM) and 10% FBS (Biowest). Cells were incubated for 48 h before fixation using Paraformaldehyde 4% and staining with Hematoxylin (Sigma). Remaining cells in upper chamber were removed with cotton tips. Cell number has been counted using ImageJ software. Western blot analysis Proteins were extracted from tissues and cells using a buffer solution with Hepes 25 mM, NaCl 400 mM, MgCl 2 1.5 mM, EDTA 200 mM, Nonidet-P40 1% supplemented with phenylmethylsulfonyl fluoride 1 mM, Na 3 VO 4 0.1 mM, NaF 0.1 mM and complete protease inhibitor cocktail (Roche Diagnostics, Meylan, France). Lysates were resolved on SDS–polyacrylamide gel electrophoresis and transferred to nitrocellulose membrane (Hybond–ECL, GE Healthcare). Membranes were incubated overnight at 4 °C with primary antibodies. Detection was performed using a peroxidase-conjugated anti-rabbit or mouse immunoglobulin G (P.A.R.I.S) and the Western Lightning System (Perkin-Elmer Life Sciences). Uncropped pictures of western blottings are available in Supplementary Fig. 14 . 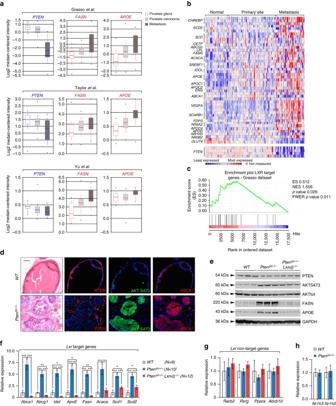Fig. 1 PTEN-loss carcinogenesis is associated with transcriptional upregulation of LXR target genes.aONCOMINE boxed plot ofPTEN,FASNandAPOEexpression levels between human prostate gland, prostate carcinoma and metastasis in various human data sets2,57,58.bHeatmap of LXR target gene signature and PTEN expression in Grasso et al.57data set.cGene Set Enrichment Analysis of LXR target gene signature based on PTEN status using Grasso et al.57data set.dHE staining and immunohistofluorescence against PTEN, AKTS473 and ABCA1 of wild type (WT) andPtenpc−/−mouse prostate tissues from 6-month-old animals.Scale bar, 100 µm. Nuclei are stained using Hoescht (blue).eWestern blot analysis of PTEN, AKTS473, AKT, FASN, APOE and GAPDH of wild type (WT),Ptenpc−/−andPtenpc−/−lxrαβ−/−mouse prostatic tissues from 6-month-old animals.f–hRelative expression of LXR targets genes, non-LXR target gene panel,Lxrα(Nr1h3) andLxrβ(Nr1h2). All data are represented as mean ± SEM and statistical analyses were performed with the Student’st-test; *p< 0.05, **p< 0.01 and ***p< 0.001. See also Supplementary Figs.1and2 Antibodies used for western blots are listed in Supplementary Table 1 . Immunochemistry Animal tissues were fixed overnight in 4% paraformaldehyde, paraffin-embedded, sectioned and stained with hematoxylin and eosin according to a standard protocol. For immunochemistry, paraffin sections were dewaxed, rehydrated, unmasked using 0.1 M citrate buffer (pH 6.0) and then incubated with primary antibodies overnight at 4 °C in a humidified chamber. Detections were performed alternatively using the NovaRED substrate kit for peroxidase (Vector Laboratories) or Alexa 488-conjugated anti-mouse IgG/Alexa 555-conjugated anti-rabbit IgG (Invitrogen). Cell nuclei were stained using Hoechst 33342 (Sigma-Aldrich). For immunofluorescence experiments, cells were seeded onto glass coverslips. Cells were fixed using 4% paraformaldehyde and permeabilized with phosphate-buffered saline (PBS)–Triton X-100 0.1% buffer. Saturation was performed using PBS bovine serum albumin 1%–FBS 1% blocking solution and incubated with respective primary antibodies. Detection was conducted using secondary antibody Alexa 488 or 555 conjugated with anti-mouse or rabbit IgG (Invitrogen). 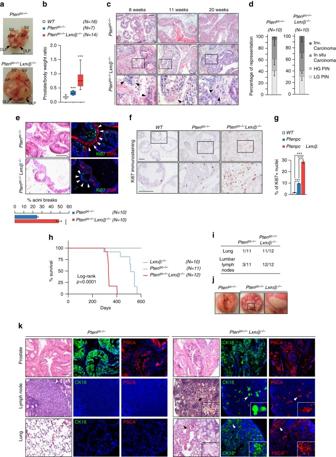Fig. 2 LXR ablation inPten-mutant mice leads to cancer progression and metastasis dissemination.aGross anatomy of representative prostates at 6 months of age. Seminal vesicles (SV), bladder (B), anterior prostate lobe (AP), dorso-lateral prostate lobe (DLP) and ventral lobe (VP).Scale bar, 1 cm.bRelative weight of prostates wild type (WT),Ptenpc−/−andPtenpc−/−lxrαβ−/−(N= 16/7/14). Statistical analyses were performed with the Student’st-test.cHE-stained sections of representative dorsal prostate (DP) at 8, 11 and 20 weeks.Scale bar, 100 µm.dHistological evaluation of dorsal lobe lesions, Low-grade PIN, high-grade PIN, in situ carcinoma or invasive carcinoma. Three distant sections from each mouse (10 mice per group) were scored (χ2= 17.27,p= 0.0006).eKi67 and SMA (smooth muscle actin) immunofluorescence performed onPtenpc−/−andPtenpc−/−lxrαβ−/−prostate specimens. Acini breaks have been quantified using following criteria: discontinuous SMA staining and presence of Ki67-positive staining in surrounding stromal compartment. Nuclei are stained using Hoescht (blue),scale bar100 µm. (N= 10 per group).fRepresentative Ki67 immunohistochemistry on prostatic tissues from each genotype,scale bar100 µm.gQuantification of Ki67-positive staining (N= 8 per group).hKaplan–Meier cumulative survival analysis showing significant decrease (p< 0.0001) in lifespan in thePtenpc−/−lxrαβ−/−compared withPtenpc−/−group. (N= 10/11/12).iRecapitulative table of metastatic phenotypes inPtenpc−/−andPtenpc−/−lxrαβ−/−animals.jGross anatomy of lungs fromPtenpc−/−vs.Ptenpc−/−lxrαβ−/−from 6-month-old mice.kHE-stained sections and immunofluorescence detection of primary tumor site (prostate), lumbar lymph nodes and lung ofPtenpc−/−andPtenpc−/−lxrαβ−/−using specific (CK18/PSCA) prostatic markers. High-magnification depicted cell arrangement within the host tissue.Scale bar, 100 µm. Nuclei are stained using Hoescht (blue). All data are represented as mean ± SEM. ***p< 0.001. See also Supplementary Figs.3,4and5 Antibodies used for immunofluorescence and immunochemistry are listed in Supplementary Table 2 . Sterol measurement Oxysterols were determined by Gas chromatography–mass spectrometry (GC–MS) using deuterium-labeled internal standards provided by Dr. Marc Poirot group [51] , [52] . In brief, for the oxysterols analysis was samples were added 10 µl BHT in ethanol (5 mg ml −1 ), 50 µl EDTA (10 mg ml −1 ) and 10 µl of ethanol containing deuterium-labeled internal standards. Alkaline hydrolysis was performed on the samples for 2 h at room temperature with stirring. Then sterols were extracted in chloroform: methanol (2:1, v/v). Solvent was evaporated under a stream of nitrogen, the sample was dissolved in 1 ml of toluene. Oxysterols were separated from cholesterol by solid phase extraction (silica cartridges 100 mg). The solvent was evaporated under a stream of nitrogen and after samples were converted to trimethylsilyl ethers by treatment with 130 µl Sylon HTP (hexamethyldisilylazane:trimethyl-chlorosilane:pyridine, 3:1:9) (Supelco, Bellafonte, PA) at 60 °C for 30 min. After incubation, the solution was evaporated under a stream of nitrogen and the residue dissolved in n -hexane and transferred to an autosampler vial. Analyses were performed on an Agilent 6890N GC equipped with a 7683 series automatic liquid sampler and interfaced with an Agilent 5973 Mass Spectrometer (Agilent Technologies, Palo Alto, CA). Separation was carried out on a 30 m capillary column (HP-5MS 30 m 0.25 mm ID, 0.25 µm thickness). Quantification of oxysterols was made by the isotope dilution method. Human data set analysis Box plots and heatmap were performed using ONCOMINE portal ( www.oncomine.org ). GSEA has been used with a list of 24 genes (e.g., genes with functionally characterized LXRE in human promoter sequence). Analysis was performed using http://www.broadinstitute.org platform with GSEA software v2.2.2 [53] , [54] . When more than one probe are available in the dataset, the probe with maximum signal was used. Mouse embryonic fibroblasts MEFs have been derived from 13.5 dpc embryos WT, Lxrα −/− , Lxrβ −/− or Lxrαβ −/− . Briefly, dorsal part of the dissected embryos have been sliced and incubated with PBS Trypsin-EDTA digestion mix (Sigma-Aldrich) at 37 °C for 45 min. Solution was homogenized using a syringe with 19 G needle and plate in DMEM (Sigma-Aldrich) supplemented with FBS 10% (Biowest), glutamine 2 mM (Sigma-Aldrich), minimal essential medium non-essential amino acids solution (Sigma-Aldrich), Streptomycin 100 µg ml −1 (Sigma-Aldrich) and Penicillin 100 µg ml −1 (Sigma-Aldrich). MEFs have been splited upon confluency until a period of massive senescence. After 2 months of culture, MEFs regrowth normally and have been considered as auto-immortalized. Cholesterol and precursors measurement To a screw-capped vial sealed with a Teflon septum, sample homogenates were added together with 250 ng D7-lathosterol, 500 ng of D6-desmosterol, 100 ng of D6-lanosterol, 20 ng D7-7α-hydroxycholesterol, D7-7β-hydroxycholesterol, D7-7ketocholesterol, D3-24S-hydroxycholesterol and D6-27-hydroxycholesterol, and 10 µg of D6-cholesterolas internal standards, 50 µl butylated hydroxytoluene (5 g l −1 ) and 50 µl EDTA (10 g l −1 ) to each vial and flushed with argon for 20 min to remove air. Alkaline hydrolysis was allowed to proceed at room temperature (22 °C) with magnetic stirring for 1 h in the presence of ethanolic 1 M potassium hydroxide solution. After hydrolysis, the sterols were extracted twice with 5 ml cyclohexane. The organic solvents were evaporated under a gentle stream of argon, and sterols and cholesterol separated by solid phase extraction with 3 ml of hexane + 0.5% isopropanol and oxysterols with 5 ml of hexane + 30% isopropanol. Sterols and oxysterols were converted into trimethylsilyl ethers with N,O -Bis(trimethylsilyl)trifluoroacetamide (BSTFA) with trimethylchlorosilane 1% (Pierce). GC–MS analysis was performed on GC equipped with an Elite column (30 m × 0.32 mm id × 0.25 mm film; Perkin Elmer, USA) and injection was performed in splitless mode and using helium (1 ml min −1 ) as a carrier gas. The temperature program was as follows: initial temperature of 180 °C was held for 1 min, followed by a linear ramp of 20 °C min −1 to 270 °C, and then a linear ramp of 5 °C min −1 to of 290 °C, which was held for 10 min. The mass spectrometer operates in the selected ion-monitoring mode. Peak integration is performed manually and sterols are quantified from selected-ion monitoring analyses against internal standards using standard curves for the listed sterols. Additional qualifier (characteristic fragment ions) ions were used for structural identification [55] , [56] . Supernatant sterol contains assay PC3 cells transfected with empty vector, pGFP–PTEN, pGFP–PTENC124A or pCMV6-HA-AKTd/n vector and/or Vitamin E, PC3 transduced with lentivirus expressing SULT2B1B, and MPEC+/+ or MPEC Pten −/− have been grown for 24 h post transfection and/or treatment in 2% LPDS. Cells RNA have been extracted and cholesterol de novo genes and LXR target genes have been analyzed as a control of treatment efficiency. Supernatants were removed, filtrated onto 0.22 µm filters and incubated with MEFs previously transfected with pCMX-UAS-Luc reporter construct and expression vector encoding pCMX-Gal4LXRα-LBD or/and pCMX-Gal4LXRβ-LBD. FBS 10% and T0901317 (1 μM) treatments have been performed as a control. Microarray analyzes Biotinylated single strand complementary DNA targets were prepared, starting from 250 ng of total RNA, using the Ambion WT Expression Kit (catalog number 4411974) and the Affymetrix GeneChip WT Terminal Labeling Kit (catalog number 900671) according to Affymetrix recommendations. Following fragmentation and end labeling, 3 μg of cDNAs were hybridized for 16 h at 45 °C on GeneChip Mouse Gene 2.0 ST arrays interrogating 35240 RefSeq transcripts and ~ 2,000 LncRNAs. The chips were washed and stained in the GeneChip Fluidics Station 450 (Affymetrix) and scanned with the GeneChip Scanner 3000 7G (Affymetrix) at a resolution of 0.7 µm. Raw data (.CEL Intensity files) were extracted from the scanned images using the Affymetrix GeneChip Command Console version 4.1.2. CEL files were further processed with Affymetrix Expression Console software version 1.4.1 to calculate probe set signal intensities using Robust Multi-array Average algorithms with default settings. Gene expression microarray data have been deposited in the GEO database with the accession number GSE96545. Reverse transcriptase–quantitative PCR For cells experiments, total RNA was isolated using Trizol reagent (Invitrogen) according to the manufacturer’s instructions. For prostates tissues, mRNA were extracted using the NucleoSpinRNAII kit (Macherey Nagel EURL, Hoerdt, France). cDNA was synthesized with MMLV-RT (Promega, Charbonnières, France) and random hexamer primers (Promega) according to the manufacturer’s instructions. Reverse transcription was performed on an Eppendorf Mastercycler (Eppendorf, Brumath, France). Four microliters of 1:20 diluted cDNA template were amplified by 0.75U of HotMaster TaqDNA polymerase (Eppendorf) using SYBR Green dye to measure duplex DNA formation on a LightCycler 480 system (Roche Diagnostics). 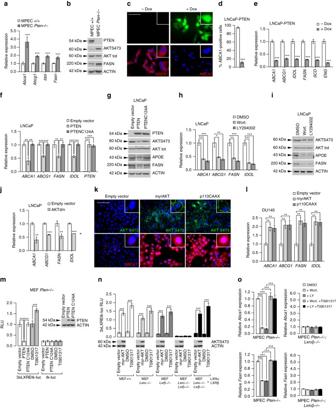Fig. 3 PTEN-status controls LXR activities in PCa cells through PI3K/AKT pathway.aRelative expression levels ofAbca1,Abcg1,Idol,Fasnand (b) PTEN, AKTS473, AKT, FASN and β-ACTIN protein accumulation levels in MPECs (mouse prostatic epithelial cells) wild-type ( + / + ) andPten−/−.cImmunofluorescence of PTEN–GFP and ABCA1 in LNCaP-PTEN inducible cell line treated with DMSO or Doxycycline (25 µM). Nuclei are stained using Hoescht (blue).Scale bar: 100 µm.dQuantitative measurement of ABCA1-positive cells has been performed.eRelative expression of LXR target genes in LNCaP-PTEN-inducible cell line treated with DMSO or Doxycycline (25 µM).f,gRelative gene expression analysis and protein accumulation of LXR targets in LNCaP cells transfected with PTEN and PTENC124A expression construct vs. empty vector.h,iRelative expression and protein accumulations of LXR targets in LNCaP cells treated with PI3K inhibitors Wortmannin (0.5 µM) or LY294002 (20 µM).jRelative accumulation ofABCA1,ABCG1,FASNandIDOLin LNCaP cells transfected with AKTd/n (dominant-negative) expression vector.kImmunofluorescence against AKTS473 and ABCA1 in DU145 transfected with myrAKT or p110CAAX (dominant-positive) expression vectors. Nuclei are stained using Hoescht (blue).Scale bar: 100 µm.lRelative accumulation ofABCA1,ABCG1,FASNandIDOLin DU145 transfected with myrAKT of p110CAAX expression vectors.mLuciferase activity measurement in MEFPten−/−transfected with 3xLXREtk-Luc reporter construct or tk-Luc construct as a control and with PTEN and PTENC124A expression construct versus empty vector.nLuciferase activity measurement in MEF + / + ,Lxrα−/−,Lxrβ−/−orLxrαβ−/−transfected with 3xLXREtk-Luc reporter construct and expression vector encoding myrAKT. T0901317 (1 µM) treatment has been performed as a control. MEFLxrαβ−/−were rescued using LXRα and LXRβ expression vectors.oAbca1andFasnrelative expression in MPECPten−/−andPten−/−lxrαβ−/−treated with Wortmannin (0.5 µM), LY294002 (20 µM) and/or T0901317 (1 µM). For whole experiments, the results represent the means ± SEM of three independent experiments; *p< 0.05; **p< 0.01; ***p< 0.001. See also Supplementary Figs6and7 Primers used for reverse transcriptase–quantitative PCR are listed in Supplementary Table 3 . Data analysis Values are expressed as means ± SEM. Statistical comparisons were performed using a two-tailed Student’s t -test or analysis of variance as indicated in the figure legends. Significance of Kaplan–Meier cumulative survival analysis was determined using Mantel–Cox log-rank test. Throughout all figures, * p < 0.05, ** p < 0.01 and *** p < 0.001. 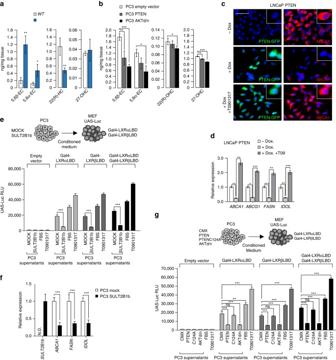Fig. 4 PTEN-loss results in an accumulation of sterols.aLevels of 5,6β-epoxy-cholesterol, 5,6α-epoxy-cholesterol, 22(R)-hydroxycholesterol and 27-hydroxycholesterol in prostatic samples from wild type (WT) (N= 4) andPtenpc−/−mice (N= 5).bLevels of 5,6β-epoxy-cholesterol, 5,6α-epoxy-cholesterol, 22(R)-hydroxycholesterol and 27-hydroxycholesterol in PC3 cells transfected with PTEN expression construct vs. empty vector.c,dImmunofluorescence of PTEN–GFP and ABCA1 proteins, and relative expression of LXR target genes in LNCaP-PTEN-inducible cell line treated with DMSO or Doxycycline (25 µM) with or without T0901317 (1 µM). Nuclei are stained using Hoescht (blue),scale bar100 µm.eLuciferase activity measurement in wild type MEF transfected with Gal4-LXRαLBD or/and Gal4-LXRβLBD and UAS-Luciferase after incubation with medium conditioned during 24 h by PC3 cells transduced with SULT2B1b or Mock construct. FBS and T0901317 are used as controls.fLXR target genes expression in PC3 cells transduced with SULT2B1b or Mock construct.gLuciferase assays in wild type MEF transfected as indicated above after incubation with medium conditioned during 24 h by PC3 cells transfected with PTEN, PTENC124A or AKTd/n expression construct versus empty vector. FBS and T0901317 are used as controls. For experimentsb–g, data are the result of three independent experiments. All the statistical analyses were performed with the Student’st-test and are represented as mean ± SEM; *p< 0.05; **p< 0.01; ***p< 0.001. See also Supplementary Figs.8,9and10 Significance was considered at p < 0.05. 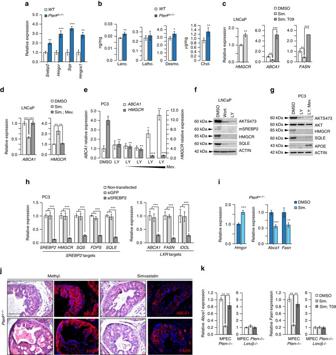Fig. 5 PTEN-loss results in an increased cholesterol de novo synthesis.aRelative accumulation ofSrebp2,Hmgcr,SqsandHmgcs1transcripts in prostate of wild type (WT) andPtenpc−/−mice. (N= 10 per group).bAccumulation of cholesterol precursors, lanosterol, lathosterol, desmosterol and cholesterol in prostatic samples from wild type (WT) (N= 4) andPtenpc−/−mice (N= 5).cqPCR analysis ofHMGCR,ABCA1andFASNexpression in LNCaP cells treated with Simvastatin (2,5 µM) alone or with T0901317 supplementation (1 µM). Experiments have been performed in three experimental replicates.dqPCR analysis ofABCA1andHMGCRexpression in LNCaP cells treated with Simvastatin (2,5 µM) alone or with mevalonate (500 µM).eqPCR analysis ofHMGCR,ABCA1andFASNexpression in PC3 cells treated with LY294002 (20 µM) alone or with increasing amounts of mevalonate (100 µM, 500 µM, 1 mM, 10 mM).fWestern blot analysis of SREBP2 cleaved form, HMGCR and SQLE respective accumulation in LNCaP cell line. AKTS473 is used to confirm Wortmannin and LY294002 treatment efficiency and β-ACTIN as a loading control.gWestern blot analysis of HMGCR, SQLE and APOE in PC3 cells treated with LY294002 (20 µM) alone or in combination with mevalonate (500 µM). AKTS473 and AKT are used to confirm Wortmannin and LY294002 treatment efficiency and β-ACTIN as a loading control.hSREBP2 and LXR target genes expression in PC3 cells transfected with siSREBP2 or siGFP as control. Experiments have been performed in three experimental replicates.iRelative expression ofHmgcr,Abca1andFasnon prostate samples from wild type mice andPtenpc−/−mice treated with vehicle (methylcellulose) or Simvastatin (40 mg kg−1).jImmunofluorescence detection of FASN and ABCA1 on prostate samples from wild type mice andPtenpc−/−mice treated with vehicle (methylcellulose,N= 6) or Simvastatin (40 mg kg−1,N= 6). Nuclei are stained using Hoescht (blue),scale bar100 µm.kqPCR analysis ofAbca1andFasnexpression on MPECPten−/−orPten−/−lxrαβ−/−treated with simvastatin alone (2,5 µM) or in combination with T0901317 (1 µM),N= 3 per group. All data are represented as mean ± SEM and statistical analyses were performed with the Student’st-test; *p< 0.05; **p< 0.01; ***p< 0.001. See also Supplementary Figs.11and12 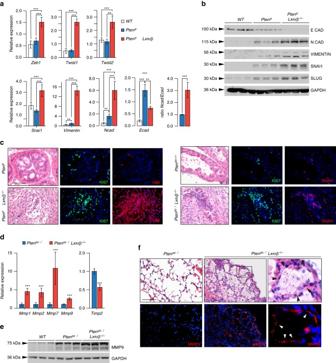Fig. 6 LXRs control invasiveness of tumor cells through upregulation of EMT and metalloproteases.a,bRelative expression and protein accumulation of EMT markers in prostate from wild type (WT),Ptenpc−/−andPtenpc−/−lxrαβ−/−mice (N= 10/7/8).cImmunofluorescence staining against EMT markers VIMENTIN and SNAI, together with Ki67. Nuclei are stained using Hoescht (blue).dRelative expression analysis of metalloproteinase genesMmp1, 2, 7, 9and negative regulatorTimp2in prostate from wild type (WT),Ptenpc−/−andPtenpc−/−lxrαβ−/−mice (N= 10 per group).eMMP9 protein accumulation in prostate from wild type (WT),Ptenpc−/−andPtenpc−/−lxrαβ−/−mice.fHistological and immunofluorescence staining for MMP9 in lung fromPtenpc−/−andPtenpc−/−lxrαβ−/−mice. White arrows indicate the positive MMP9 staining surrounded metastatic cells in contact with matrix. Asterisks identify metastatic cells and black arrows the surrounded pneumocytes. Nuclei are stained using Hoescht (blue). All data are represented as mean ± SEM and statistical analyses were performed with the Student’st-test; **p< 0.01; ***p< 0.001. See also Supplementary Fig.13 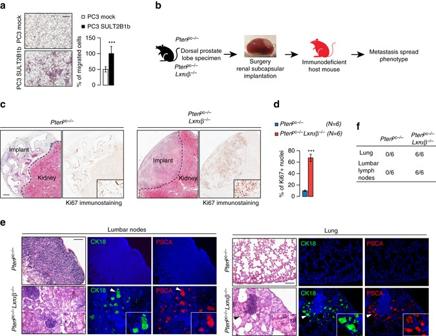Fig. 7 LXRs downregulate intrinsic invasiveness properties of PTEN-negative tumor cells.aBoyden chamber assays performed using PC3 cells transduced with SULT2B1b or Mock construct. Migrated cells are stained with hematoxylin staining (N= 8),scale bar100 µm.bDescription for renal subcapsular implantation in immunocompromized host mice (Nude mice) of prostate specimen fromPtenpc−/−andPtenpc−/−lxrαβ−/−mice.c,dRepresentative histological features (HE) and Ki67 staining of implant after 1 month of growth, and quantification of Ki67-positive cells fromPtenpc−/−(N= 6) andPtenpc−/−lxrαβ−/−(N= 6) grafts on Nude mice,scale bar100 µm.eEvaluation of metastatic dissemination on lumbar lymph nodes and lung using prostatic markers CK18 and PSCA in grafted nude mice (N= 6 per group). Nuclei are stained using Hoescht (blue),scale bar100 µm.fRecapitulative table of metastatic phenotype in lungs and lumbar lymph nodes of grafted Nude mice. All data are represented as mean ± SEM and statistical analyses were performed with the Student’st-test; ***p< 0.001 Data availability Gene expression microarray data have been deposited in the GEO database ( http://www.ncbi.nlm.gov/geo ) with the accession number GSE96545. The authors declare that all the other data supporting the findings of this study are available within the article and its Supplementary Information Files and from the corresponding authors on reasonable request.